Two-colour spin noise spectroscopy and fluctuation correlations reveal homogeneous linewidths within quantum-dot ensembles ‘Spin noise spectroscopy’ is an optical technique for probing electron and hole spin dynamics that is based on detecting their intrinsic fluctuations while in thermal equilibrium. Here we show that fluctuation correlations can be further exploited in multi-probe noise studies to reveal information that in general cannot be accessed by conventional linear optical spectroscopy, such as the underlying homogeneous linewidths of individual constituents within inhomogeneously broadened systems. This is demonstrated in singly charged (In,Ga)As quantum-dot ensembles using two weak probe lasers: When the lasers have similar wavelengths, they probe the same quantum dots in the ensemble and show correlated spin fluctuations. In contrast, mutually detuned probe lasers measure different subsets of quantum dots, giving uncorrelated fluctuations. The noise correlation versus laser detuning directly reveals the quantum dot homogeneous linewidth even in the presence of a strong inhomogeneous broadening. Such noise-based correlation techniques are not limited to semiconductor spin systems, but are applicable to any system with measurable intrinsic fluctuations. Inhomogeneous broadening is ubiquitous in the physical, chemical and materials sciences, occurring whenever a collection of nominally equivalent constituents differ in size, shape, composition, conformation and/or local environment. Notable examples in nanoscale materials include ensembles of nanocrystals, quantum dots, nanotubes or molecules [1] , [2] , [3] . In optically active systems, such broadening typically leads to a spread of the constituents’ fundamental absorption or emission energies over an inhomogeneously broadened band of spectral width γ inh , which can be orders of magnitude larger than the underlying homogeneous linewidth γ h of the individual constituents themselves [3] , [4] , [5] , [6] , [7] , [8] . Usually, however, γ h is the essential quantity of interest, since γ h directly reveals (or at least constrains) the fundamental relaxation rates and coherence times of the system, which are the crucial parameters for many applications. Unfortunately, γ h is generally inaccessible in inhomogenously broadened ensembles using conventional low-power/linear optical spectroscopic techniques, which typically measure time- and ensemble-averaged response functions (such as absorption, photoluminescence, polarization, etc). To circumvent this limitation, various nonlinear optical methods have been very successfully developed over the years to extract γ h from inhomogeneously broadened ensembles; examples include spectral-hole burning [9] , [10] and four-wave mixing methods [11] , [12] , [13] , [14] , [15] , which necessarily rely on the excitation and nonlinear optical response of the material. In parallel, a multitude of optical techniques for isolating and measuring single particles [3] , [4] , [5] , [6] , [7] , [8] have also been developed to get around the problem of inhomogeneous broadening in ensemble studies. In this broader context, it is also worth highlighting prior efforts to harness intensity correlations in ensemble photoluminescence as a means to infer γ h (refs 16 , 17 ). In this work we develop a novel low-power optical technique—two-colour spin noise spectroscopy—and demonstrate that it can be used to reveal the underlying homogeneous linewidth γ h of the individual constituents that make up an otherwise inhomogeneously broadened ensemble. Specifically we apply these methods to reveal γ h of singly charged (In,Ga)As quantum dots (QDs) within an inhomogeously broadened QD ensemble. Importantly, this optical technique operates in the linear/low-power regime and does not rely on any excitation or nonlinear response of the system. The key point is that this technique is not based on conventional time-averaged response functions, but rather is based on the intrinsic and random fluctuation properties of the system—in this case, spin fluctuations. In particular, it exploits the fact that spin fluctuations from different QDs in the ensemble are uncorrelated in time. By measuring the degree of correlation between two independent noise probes (two probe lasers detuned from each other), we reveal the underlying homogeneous absorption linewidth, γ h , of positively charged QDs in an ensemble measurement—information that is generally inaccessible to conventional linear spectroscopy. Spin noise of QDs using a single probe laser Optical spin noise spectroscopy (SNS) is a powerful and relatively new technique for probing the dynamics of electron and/or hole spins, that is based on measuring their intrinsic fluctuations while they remain unperturbed and in thermal equilibrium [18] , [19] , [20] . This approach, though nonstandard, is nonetheless assured by the fluctuation-dissipation theorem, which relates linear response functions to the frequency spectrum of intrinsic fluctuations [21] . In a typical SNS experiment, random spin fluctuations δS z ( t ) in an equilibrium sample impart Faraday rotation (optical polarization rotation) fluctuations δθ ( t ) on a probe laser, which can be measured with high sensitivity. In the frequency domain, the peak positions, widths and amplitudes of this Faraday rotation (FR) noise reveal the detailed dynamical properties of the spins such as g -factors, coherence times and relaxation rates—without (in principle) ever exciting or pumping the spin system itself. This latter appealing aspect arises because spin detection via FR depends on the system’s dispersive indices of refraction (rather than absorption), and in many systems it can form the basis for continuous quantum nondemolition measurement [22] , [23] . Optical SNS has been applied to alkali vapours [18] , electrons in bulk n -type GaAs [24] , [25] , quantum well microcavities [26] and recently to electron and hole spins in (In,Ga)As QD ensembles [27] , [28] . In all SNS studies reported to date, a single probe laser was used to detect the intrinsic spin fluctuations of the system. For the studies of QD ensembles [27] , [28] , this probe laser was tuned in wavelength to lie directly within the inhomogeneously broadened absorption/photoluminescence band of the ensemble. Because individual QDs within the ensemble have very narrow homogeneous linewidths γ h at low temperature [4] , [5] , [6] , [7] , [8] , the probe laser is particularly sensitive to spin fluctuations from those singly charged QDs having charged exciton (trion) optical transition energies close to the laser energy. Consider, as depicted in Fig. 1a , an inhomogeneously broadened QD ensemble and two singly charged dots (QDA and QDB) with different trion transition energies within this ensemble. Per the usual optical selection rules for spins in III–V or II–VI semiconductors [7] , [29] , individual QDs within this ensemble exhibit spin-dependent absorption spectra for right- and left-circularly polarized light ( α R,L , assumed to be Lorentzian) that depend on the orientation of the resident spin. 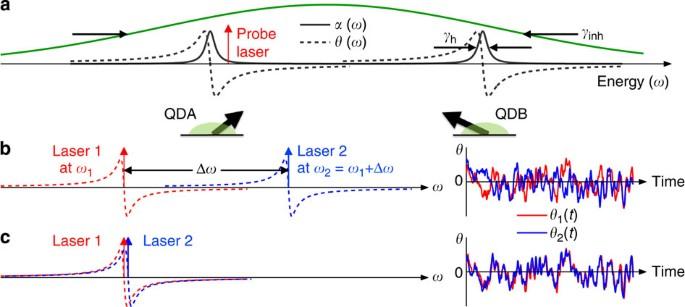Figure 1: Correlated and uncorrelated spin fluctuations in inhomogeneously broadened QD ensembles. (a) Illustrations depicting the inhomogeneously broadened absorption band of a QD ensemble (green line), along with the homogeneously broadened absorption and associated Faraday rotation spectra [α(ω) andθ(ω)] of two representative singly charged QDs in the ensemble (QDA and QDB). The probe laser that is shown is primarily sensitive to fluctuations of the spin in QDA, but not QDB. (b) Cartoon showing two probe lasers at photon energiesω1andω2. The dotted lines depict the Faraday rotation (FR) sensitivity of each laser to spin fluctuations in QDs at energyω, which has the same functional form asθ(ω) (note that the probe lasers are not sensitive to spin noise from QDs exactly on resonance, becauseθ(ω) is an odd function). Here, the two lasers are well separated in energy (Δω≫γh), and therefore they are sensitive to different subsets of QDs, so that the FR noise on the two lasers [θ1(t) andθ2(t)] are largely uncorrelated in time. (c) The same, but for the case of small laser detuning (Δω≤γh). Here, the two lasers probe predominantly the same dots and FR noise is correlated, giving larger measured noise power ‹[θ1(t)+θ2(t)]2›. For example, Figure 1: Correlated and uncorrelated spin fluctuations in inhomogeneously broadened QD ensembles. ( a ) Illustrations depicting the inhomogeneously broadened absorption band of a QD ensemble (green line), along with the homogeneously broadened absorption and associated Faraday rotation spectra [ α ( ω ) and θ ( ω )] of two representative singly charged QDs in the ensemble (QDA and QDB). The probe laser that is shown is primarily sensitive to fluctuations of the spin in QDA, but not QDB. ( b ) Cartoon showing two probe lasers at photon energies ω 1 and ω 2 . The dotted lines depict the Faraday rotation (FR) sensitivity of each laser to spin fluctuations in QDs at energy ω , which has the same functional form as θ ( ω ) (note that the probe lasers are not sensitive to spin noise from QDs exactly on resonance, because θ ( ω ) is an odd function). Here, the two lasers are well separated in energy (Δ ω ≫ γ h ), and therefore they are sensitive to different subsets of QDs, so that the FR noise on the two lasers [ θ 1 ( t ) and θ 2 ( t )] are largely uncorrelated in time. ( c ) The same, but for the case of small laser detuning (Δ ω ≤ γ h ). Here, the two lasers probe predominantly the same dots and FR noise is correlated, giving larger measured noise power ‹[ θ 1 ( t )+ θ 2 ( t )] 2 ›. Full size image if the resident spin has projection ‘spin-up’ along the probe laser , while α R and α L are swapped for opposite spin projection. Here, ω is the photon energy, ω k is the energy of the charged exciton transition of the QD in question, and γ h is its homogeneous absorption linewidth. The Faraday rotation, θ , that is imparted to a probe laser by this spin-dependent optical transition scales as the difference between the associated indices of refraction, n R and n L : Therefore when the resident spin in a QD fluctuates randomly in time, θ ( t ) also fluctuates. In thermal equilibrium and in zero magnetic field, its time average is of course zero (‹ θ ( t )›=0), but its variance ‹ θ 2 ( t )›—the FR noise power—is nonzero and is peaked at photon energies ± γ h /2 away from the QD resonance, and decays as | ω − ω k | −2 for large detuning. (Note also that spin fluctuations induce no FR noise exactly on resonance when ω = ω k , because θ is an odd function). Therefore the probe laser depicted in Fig. 1a , which has photon energy close to the QDA trion resonance, is much more sensitive to spin (FR) fluctuations from QDA than from QDB. Two-colour spin noise spectroscopy We exploit this spectral selectivity, and also the fact that fluctuations of spins in different dots are nominally uncorrelated in time, to directly obtain γ h in an ensemble measurement, using a low-intensity (linear) optical experiment based on spin noise. Specifically, we use two different probe lasers (‘1’ and ‘2’) that are tuned within the broad absorption band of the QD ensemble, and measure the degree of correlation between the FR fluctuations that are imparted on the two lasers [ θ 1 ( t ) and θ 2 ( t )]. The two co-propagating probe lasers are incident on the same photodetector, and the total measured FR is just the sum θ 1 ( t )+ θ 2 ( t ). The variance of the FR noise (that is, the measured noise power) is therefore Figure 1b depicts the two detuned probe lasers, and the accompanying dotted lines illustrate how much FR is imparted on that probe laser due to QDs at energy ω . If, as shown, the detuning Δ ω between the two lasers is large (Δ ω ≫ γ h ), then each laser is sensitive to a different and independent subset of fluctuating spins, and θ 1 ( t ) and θ 2 ( t ) are uncorrelated and add incoherently (that is, the cross-term in equation (3) averages to zero). In contrast, if Δ ω ≤ γ h (see Fig. 1c ), then the lasers measure predominantly the same QDs, θ 1 ( t )≈ θ 2 ( t ) and the FR fluctuations are correlated, giving larger measured noise power. The two-colour spin noise experiment is depicted in Fig. 2a . The low-power outputs from two tunable continuous-wave probe lasers (1 and 2, each having <10 MHz linewidth) are combined and launched through a single-mode polarization-maintaining fibre to ensure spatial overlap. The light is linearly polarized and focused weakly through an ensemble of singly charged QDs. Stochastic fluctuations of the hole spins in the QDs generate FR fluctuations θ ( t )= θ 1 ( t )+ θ 2 ( t ) on the transmitted probe beam, which are measured with balanced photodiodes. The output voltage V ( t ) ∝ θ ( t ) is continuously digitized and Fourier-transformed in real time [27] to obtain the noise power density spectrum (shown here in units of V 2 Hz −1 ). Mechanical shutters control whether the probe beam is composed of laser 1, 2 or both. The samples are lightly p -type (In,Ga)As/GaAs QDs grown by molecular beam epitaxy (see Methods). Owing to statistical variations in QD size and composition, the ensemble PL spectrum is strongly inhomogeneously broadened ( γ inh ~20 meV), and is peaked at ~1.385 eV (895 nm). 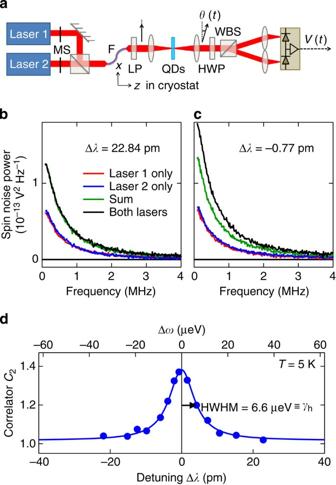Figure 2: Measuring the two-colour spin noise correlatorC2(Δω) and QD homogeneous linewidthγh. (a) Experimental schematic: narrowband probe lasers 1 and 2 are combined in a single-mode polarization-maintaining fibre (F). The probe light is weakly focused through the ensemble of singly charged QDs, where hole spin fluctuations impart FR noise on the transmitted light, which is measured by balanced photodiodes. Here, MS are mechanical shutters, LP is a linear polarizer, HWP is a half-wave plate and WBS is a Wollaston beam splitter. HWP can be replaced by a quarter-wave plate to measure ellipticity noise. (b,c) Raw spin noise power spectra for the case of large and small laser detuning (Δω>γhand Δω<γh), giving uncorrelated and correlated spin noise, respectively;T=5 K. The red and blue spectra were detected using only laser 1 or laser 2, respectively. The green trace is their mathematical sum. The black trace was measured with both lasers on simultaneously. (d) Two-colour spin noise correlatorC2as a function of the detuning between the probe lasers. The solid line is a Lorentzian fit, and its HWHM reveals the underlying homogeneous linewidthγhof the QDs. Figure 2: Measuring the two-colour spin noise correlator C 2 (Δ ω ) and QD homogeneous linewidth γ h . ( a ) Experimental schematic: narrowband probe lasers 1 and 2 are combined in a single-mode polarization-maintaining fibre (F). The probe light is weakly focused through the ensemble of singly charged QDs, where hole spin fluctuations impart FR noise on the transmitted light, which is measured by balanced photodiodes. Here, MS are mechanical shutters, LP is a linear polarizer, HWP is a half-wave plate and WBS is a Wollaston beam splitter. HWP can be replaced by a quarter-wave plate to measure ellipticity noise. ( b , c ) Raw spin noise power spectra for the case of large and small laser detuning (Δ ω > γ h and Δ ω < γ h ), giving uncorrelated and correlated spin noise, respectively; T =5 K. The red and blue spectra were detected using only laser 1 or laser 2, respectively. The green trace is their mathematical sum. The black trace was measured with both lasers on simultaneously. ( d ) Two-colour spin noise correlator C 2 as a function of the detuning between the probe lasers. The solid line is a Lorentzian fit, and its HWHM reveals the underlying homogeneous linewidth γ h of the QDs. Full size image Figure 2b shows the measured power spectra of hole spin noise for the case of large detuning between probe lasers (Δ λ =22.84 pm, or Δ ω =35.36 μeV). The red and blue noise spectra were acquired using the individual lasers 1 and 2 alone. The noise spectra are Lorentzian with ~500 kHz half-width, indicating long hole spin relaxation times of ~300 ns, in agreement with previous (single-probe) noise studies of similar QD ensembles [28] . The green spectrum is just the mathematical sum of these two single-probe measurements. The black spectrum is the spin noise acquired using both lasers 1 and 2 simultaneously. Here, this black trace overlaps almost exactly with the green, indicating that in this case the FR fluctuations on the two lasers are uncorrelated: the noise power with both lasers is simply the sum of the noise power from the two individual probe lasers because the interference term in equation (3) vanishes. In marked contrast, Fig. 2c shows the case for small detuning between the probe lasers (Δ λ =−0.77 pm, or Δ ω =−1.19 μeV). Here, the spin noise power measured with both lasers simultaneously is greater than the sum of the noise power measured by lasers 1 and 2 individually, indicating that the FR noise encoded on the two probe lasers is at least partially correlated such that the interference term in equation (3), ‹ θ 1 ( t ) θ 2 ( t )›, exceeds zero. Two-colour spin noise correlator We define the two-colour spin correlator as expressed here as a function of the photon energy ω 1 of probe laser 1 and the detuning Δ ω between lasers 1 and 2. Here, P 1 ( ω 1 ) and P 2 ( ω 2 = ω 1 +Δ ω ) are the total spin noise power measured by individual probe lasers 1 and 2, respectively (computed via the area under the measured noise spectra in Fig. 2b,c ). P both ( ω 1 ,Δ ω ) is the total spin noise power measured using both lasers simultaneously. Following equation (3), we can therefore expect the two-colour spin correlator C 2 =1 if the noise on the two lasers is uncorrelated, but increases to 2 when the noise is perfectly correlated and θ 1 ( t )= θ 2 ( t ). Figure 2d shows the measured C 2 versus detuning Δ ω . It is clearly peaked at Δ ω =0 as expected, and falls rapidly to unity as |Δ ω | increases. It fits very well to a Lorentzian function with a very narrow half-width at half-maximum (HWHM) of 4.27 pm, or 6.6 μeV. As shown immediately below, the key point of two-colour spin noise spectroscopy is that the half-width of C 2 (Δ ω ) directly reveals the underlying homogeneous absorption linewidth γ h of the singly charged QDs in the ensemble. It is straightforward to show that C 2 (Δ ω ) is expected to exhibit a Lorentzian shape with HWHM equal to γ h . First, note that the total FR noise power detected by a single probe laser at energy ω i is given by integrating up the FR noise power ‹ θ 2 ( t )› generated by all the QDs (at energies ω k ) in the ensemble: where θ i ( ω i , ω k ) has the same form as in equation (2), and ρ ( ω k ) is the inhomogeneously broadened distribution of QD energies characterized by γ inh . Effectively, this corresponds to integrating the square of the dotted red or blue curves in Fig. 1b , weighted by ρ ( ω k ). As discussed earlier, most of the noise power comes from those QDs with resonances close to the probe laser. When both lasers probe the QDs simultaneously (at ω 1 and ω 2 = ω 1 +Δ ω ), the total spin noise power is which corresponds to integrating the square of the sum of the dotted red and blue lines in Fig. 1b,c . With both lasers tuned within the inhomogeneously broadened ensemble, and since γ inh greatly exceeds both γ h and typical detunings Δ ω , ρ ( ω k ) can be approximated by a uniform distribution [ ρ ( ω k )~1] and C 2 can be calculated analytically: which is a Lorentzian with HWHM= γ h . (We note that if the lasers are tuned far outside of the inhomogeneous absorption band then C 2 (Δ ω ) is expected to be constant, a scenario that will be discussed and modelled later). Thus, using only low-power continuous-wave probe lasers and performing passive measurements, the homogeneous linewidth γ h of singly charged QDs is revealed in an ensemble measurement. Crucially, this is made possible because we measure fluctuations and correlations of the (spin-dependent) optical response function θ ( ω ) of the QDs due to spin noise, rather than conventional time-averaged linear responses. We emphasize that this measurement is free from inhomogeneous broadening effects that arise not only from a spread of QD sizes and compositions, but also from effects of spectral wandering of the QD resonances due to charge fluctuations. The measured value ( γ h =6.6 μeV) is in rather good agreement with recent nonlinear four-wave mixing studies [15] of very similar positively charged (In,Ga)As QD ensembles ( γ h =8±2 μeV at 10 K) and also with absorption measurements of individual positively charged InGaAs QDs ( γ h ~5 μeV at 4.2 K in refs 6 , 7 , and γ h ~2 GHz ≡8.2 μeV at 5 K in ref. 30 ). It is less than γ h inferred from coherent control studies of hole qubits in single InAs-based QDs (6.7 GHz ≡27 μeV at 1.6 K) in ref. 31 , but in all cases the different QD growth and device fabrication conditions make direct comparisons difficult. We note that both the principle and the technique of two-colour spin noise spectroscopy—as well as the information obtained—are essentially different than the methods for ‘optical spectroscopy of spin noise’ discussed recently by Zapasskii et al. [32] , who describe how single-probe SNS measurements can be used to tell the difference between homogeneous and inhomogeneously broadened lines, or to infer whether the ratio γ inh / γ h is changing in response to some external parameter like temperature. Moreover, ref. 32 concerns exclusively single-probe SNS experiments (not multi-probe), and measurements of noise power only (not correlations). Most importantly, direct measurements of γ h are not possible, in contrast to the case here. Control experiment on n -GaAs To validate this two-colour noise technique, Fig. 3 shows a control experiment on bulk n -type GaAs. As shown in earlier studies [25] , [33] , spin fluctuations of electrons in the conduction band of n -GaAs generate FR fluctuations that can be detected at photon energies far below the low temperature GaAs bandgap (for example, at sub-gap wavelengths from 830–900 nm), owing to the long tails of the dispersive indices of refraction (see inset). Importantly, FR noise detected at these low energies derives primarily from the same fluctuating electron spins in the conduction band, independent of probe laser wavelength. Thus, we expect correlated noise and C 2 (Δ ω )=2 in a two-colour noise experiment on n -GaAs, independent of Δ ω . Exactly this behaviour was observed and confirmed, as shown in Fig. 3 . Note that this experiment corresponds to a situation where both probe lasers are tuned well outside of any inhomogeneously broadened absorption band, a scenario that is discussed and modelled later in the paper. 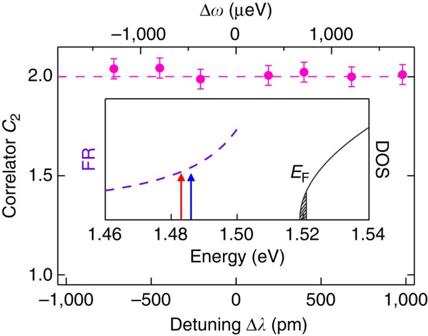Figure 3: Control experiment onn-type bulk GaAs (n=3.7 × 1016cm−3),T=10 K. Here the spin noise of electrons at the bottom of the conduction band can be probed at photon energies well below the GaAs bandgap (ω1~1.485 eV). The correlatorC2is always 2, independent of the detuning Δω. The error bars represent theχ2uncertainty when fitting the raw noise data to a Lorentzian function. The inset depicts the density of states (DOS) in GaAs, the Fermi level of the electron sea (EF), and the FR that is induced at sub-gap energies when these electrons are polarized (dashed line). Figure 3: Control experiment on n -type bulk GaAs ( n =3.7 × 10 16 cm −3 ), T =10 K. Here the spin noise of electrons at the bottom of the conduction band can be probed at photon energies well below the GaAs bandgap ( ω 1 ~1.485 eV). The correlator C 2 is always 2, independent of the detuning Δ ω . The error bars represent the χ 2 uncertainty when fitting the raw noise data to a Lorentzian function. The inset depicts the density of states (DOS) in GaAs, the Fermi level of the electron sea ( E F ), and the FR that is induced at sub-gap energies when these electrons are polarized (dashed line). Full size image Although Fig. 2d shows that C 2 (Δ ω ) for the QD ensemble exhibits the anticipated Lorentzian line shape and reveals the expected γ h , we note that its peak value is only ~1.4, which is less than the value of 2 that was observed in the n -GaAs control sample and which is expected from equation (7). This is because the probe lasers are tuned directly within the absorption band of the QD ensemble, and are therefore unavoidably pumping those QDs that are resonant with the lasers. In this regime the probe lasers cannot be considered completely non-perturbing, as evidenced by the fact that the measured spin noise density (in units of V Hz −1/2 ) increases only sublinearly with laser intensity I (and the spin noise power density in units of V 2 Hz −1 increases less than quadratically with I ). For the very narrowband lasers used in these studies (<10 MHz), independent experiments confirm that the measured noise power increases as ~ I 1.5 instead of I 2 . This is consistent with the peak value of the correlator C 2 (Δ ω ~0) measured in Fig. 2d (2 1.5 /2≈1.4). Temperature and intensity dependence It is well established from optical studies of single QDs and also from nonlinear optical studies of QD ensembles that the measured γ h is strongly dependent on the intensity of the probing light [8] , [9] . 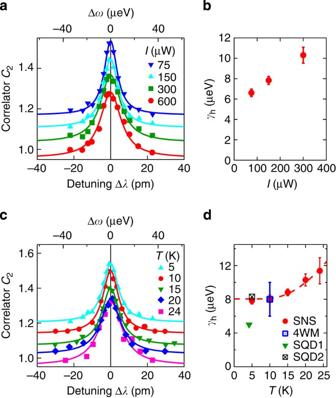Figure 4: Measuring the two-colour spin noise correlatorC2(Δω) and homogeneous linewidth γhversus laser intensity and temperature. (a)C2(Δω) at different probe laser intensitiesIat 5 K (vertically offset for clarity). (b) The corresponding homogeneous linewidths of the QDs. (c)C2(Δω) at various temperatures (vertically offset).I=150 μW. (d) The extracted homogeneous linewidthγh(red dots). The dotted line is a fit to the data following the model in ref.12. The error bars representχ2uncertainty when fitting the correlator data inaandcto Lorentzians. Also shown isγhdetermined by nonlinear four-wave mixing measurements of positively charged exciton transitions (blue square) on similar (In,Ga)As QD ensembles at 10 K (ref.15), and from absorption studies6,30of hole-doped single QDs (triangle, black square). Figure 4a,b explores the influence of probe laser intensity I on the two-colour noise correlator C 2 (Δ ω ) at 5 K. The inferred γ h increases with I , similar to past studies [8] , [9] , likely due to the resonant QD pumping effects and excitation-induced broadening discussed above. In the limit of zero laser intensity, these data suggest γ h ~6 μeV for the positively charged trion transition in these QDs, which is consistent with prior results [6] , [7] , [15] , [30] as discussed above. Figure 4: Measuring the two-colour spin noise correlator C 2 (Δ ω ) and homogeneous linewidth γ h versus laser intensity and temperature. ( a ) C 2 (Δ ω ) at different probe laser intensities I at 5 K (vertically offset for clarity). ( b ) The corresponding homogeneous linewidths of the QDs. ( c ) C 2 (Δ ω ) at various temperatures (vertically offset). I =150 μW. ( d ) The extracted homogeneous linewidth γ h (red dots). The dotted line is a fit to the data following the model in ref. 12 . The error bars represent χ 2 uncertainty when fitting the correlator data in a and c to Lorentzians. Also shown is γ h determined by nonlinear four-wave mixing measurements of positively charged exciton transitions (blue square) on similar (In,Ga)As QD ensembles at 10 K (ref. 15 ), and from absorption studies [6] , [30] of hole-doped single QDs (triangle, black square). Full size image It is also well known that γ h broadens with increasing temperature in epitaxial QDs due to interactions with phonons. Figure 4c,d shows the temperature dependence of C 2 (Δ ω ) and γ h . γ h is nearly constant below 10 K, but increases at higher temperatures. This overall trend agrees very well with available reported data on the temperature dependence of exciton linewidths in undoped but otherwise very similar (In,Ga)As QDs [12] , [13] , and also on interfacial GaAs QDs [14] , both of which were measured by nonlinear ultrafast four-wave mixing techniques. For a direct visual comparison, Fig. 4d also plots γ h determined from other studies of positively charged (In,Ga)As QDs discussed above [6] , [7] , [15] , [30] , with which our results are also in quite reasonable agreement, confirming the viability and utility of this low-power noise-based optical technique. Ellipticity noise We also show that measurements of γ h are possible by measuring ellipticity fluctuations imparted on the transmitted probe light (instead of FR fluctuations). Whereas spin fluctuations induce FR noise via the dispersive real part of the QD dielectric function (that is, the indices of refraction n R,L ), ellipticity noise is associated with fluctuations of the imaginary part (that is, the absorption α R,L ). Ellipticity and FR noise are linked via Kramers–Kronig relations and are therefore related. By replacing the half-wave plate in Fig. 2a with a quarter-wave plate, ellipticity noise is measured. 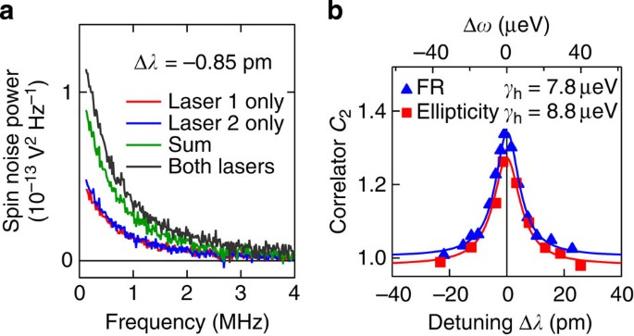Figure 5: Spin noise can also be measured via ellipticity fluctuations of the probe laser(s). (a) Raw ellipticity noise power spectra at 5 K,I=150 μW. (b) Directly comparingC2(Δω) from FR and ellipticity spin noise measurements, using the same probe laser power. Figure 5 shows raw ellipticity noise power from these QDs at 5 K, along with C 2 (Δ ω ). Following a similar analysis, the ellipticity correlator is found to have the same functional form as in equation (7), that is, a Lorentzian line shape with HWHM= γ h . For a given laser intensity I , we find that γ h obtained via ellipticity noise is slightly larger than γ h determined from FR noise ( Fig. 5b ), a likely consequence of the excitation-induced broadening discussed above and the fact that ellipticity is by definition more sensitive to absorption and therefore to QDs exactly on resonance with the probe lasers. Figure 5: Spin noise can also be measured via ellipticity fluctuations of the probe laser(s). ( a ) Raw ellipticity noise power spectra at 5 K, I =150 μW. ( b ) Directly comparing C 2 (Δ ω ) from FR and ellipticity spin noise measurements, using the same probe laser power. Full size image Modelling the two-colour noise correlator Finally, Fig. 6 shows model calculations of the two-colour noise correlator C 2 over a broad range of the two probe laser energies ω 1 and ω 2 , using equations (4, 5, 6). For simplicity we consider an idealized inhomogeneously broadened Gaussian absorption band with γ inh =100 γ h . In the usual case where the probe lasers detect spin fluctuations via Faraday rotation, Fig. 6a shows that when ω 1 and/or ω 2 is tuned within this broad inhomogeneous band, the spin noise is everywhere uncorrelated ( C 2 =1) except along the thin diagonal line corresponding to ω 1 ~ ω 2 (more specifically, when Δ ω ≲ γ h ). Expanding this region ( Fig. 6b ), this thin band has a half-width equal to γ h , as expected from equation (7) and as experimentally observed in Figs 2 and 4 . Interestingly, however, when both ω 1 and ω 2 lie well outside this broad absorption band, then neither probe laser is preferentially sensitive to nearly resonant QDs (because there are no QDs at the probe energies). In this case, both lasers are sensitive to the total FR fluctuations from the entire ensemble, and their fluctuations will be correlated ( C 2 =2) independent of Δ ω (or anti-correlated giving C 2 =0 if the lasers are on opposite ‘sides’ of this idealized band, because θ ( ω ) is an odd function). This was precisely the case for the two-colour spin noise measurement on the n -type GaAs control sample shown in Fig. 3 . A similar modelling can be performed for the case when spin fluctuations are measured via ellipticity noise, as shown in Fig. 6c,d and as experimentally observed in Fig. 5 . (Note, however, that although C 2 can be calculated for all ( ω 1 , ω 2 ), ellipticity noise must generally be measured within the absorption band because otherwise the noise signals themselves become extremely small.) 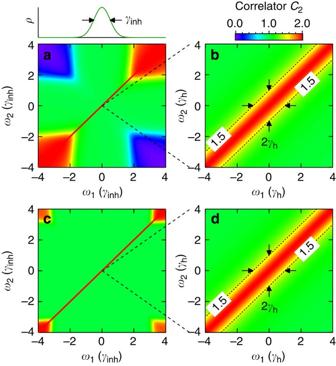Figure 6: Modelling the two-colour spin noise correlatorC2as a function of the two probe laser energiesω1andω2(horizontal and vertical axis, respectively). We consider an inhomogeneously broadened Gaussian band withγinh=100γh. (a) The case when FR noise is detected; see text for details. (b) An expanded view along the diagonal whereω1~ω2(note change in scale). (c,d) The case when ellipticity noise is detected. Figure 6: Modelling the two-colour spin noise correlator C 2 as a function of the two probe laser energies ω 1 and ω 2 (horizontal and vertical axis, respectively). We consider an inhomogeneously broadened Gaussian band with γ inh =100 γ h . ( a ) The case when FR noise is detected; see text for details. ( b ) An expanded view along the diagonal where ω 1 ~ ω 2 (note change in scale). ( c , d ) The case when ellipticity noise is detected. Full size image We have introduced and demonstrated the new optical technique of two-colour spin noise spectroscopy. Despite being a low-power optical method that does not rely on excitation, pumping or perturbation of the ensemble, it can directly reveal the underlying homogeneous linewidths of QDs that are otherwise obscured in strongly inhomogeneously broadened optical spectra. This is because these methods are based on fluctuations and correlations, rather than on measurement of the standard time-averaged response functions that are measured by conventional linear optical spectroscopy. Though demonstrated here for the specific case of semiconductor QDs and spin fluctuations, the general principle should be broadly applicable to many classes of systems and materials in which intrinsic fluctuations can be detected—and may prove especially attractive for those systems where the individual constituents cannot easily be isolated, or for which intense nonlinear perturbation is undesired. Moreover, these noise-based techniques can equally well be applied to—and have great promise for—studies of correlations in interacting systems, such as coupled quantum-dot or nanocrystal systems, spin-exchange interactions in atomic gases or spin–spin interactions in chemical and biological systems. A further interesting extension of these ideas is to measure not only temporal but also spatial correlations of systems exhibiting collective excitation (for example, magnon, plasmon or polariton systems), by two or more probes with tunable spatial separation [34] . Quantum dot samples Self-assembled InAs/GaAs QDs were grown by molecular beam epitaxy on (001) GaAs substrates, and then thermally annealed at 940 °C for 30 s. Annealing interdiffuses indium and gallium and thus increases the size of the QDs and decreases the depth of the confining potential, blue-shifting the QD absorption band to ~900 nm. The sample contains 20 layers of QDs, separated by 60 nm GaAs barriers, with QD density of 10 10 cm −2 in each layer. The sample is weakly p -type due to background carbon doping; we estimate that ~10% of the QDs contain a single resident hole. The measured spin noise arises from stochastic spin fluctuations of the resident holes trapped in the singly charged subset of QDs. The control experiment was carried out on a bulk n -GaAs wafer with electron density 3.7 × 10 16 cm −3 . Experimental setup The samples are mounted on the cold finger of a liquid helium optical cryostat. All noise data shown were acquired at zero magnetic field, following refs 25 , 27 . Two tunable narrowband continuous-wave diode lasers (from Toptica and New Focus, both with <10 MHz linewidth) are tuned in wavelength near the centre of the inhomogeneously broadened photoluminescence/absorption spectrum of the QD ensemble. Typical focused spot sizes are ~25 μm (~10 6 QDs lie within the spot, ~10 5 of which are charged), with ~100 μW power from each laser. In all the data shown, the first laser remains at a fixed wavelength of 896.3 nm (1.387 eV); the second one is detuned from the first one by Δ ω . γ h did not vary appreciably for different values of ω 1 . For the control experiment on bulk n -GaAs, we use two continuous-wave Ti:sapphire lasers (from Coherent). The lasers were tuned ~30 meV below the low-temperature absorption edge of bulk GaAs ( E gap =1.515 eV or 818 nm). The spin noise signal is continuously digitized and processed by a field-programmable gate array [27] to obtain the spin noise power spectrum; each data point requires a few minutes of signal averaging. How to cite this article: Yang, L. et al. Two-colour spin noise spectroscopy and fluctuation correlations reveal homogeneous linewidths within quantum-dot ensembles. Nat. Commun. 5:4949 doi: 10.1038/ncomms5949 (2014).